A role for calpain-dependent cleavage of TDP-43 in amyotrophic lateral sclerosis pathology Both mislocalization of TDP-43 and downregulation of RNA-editing enzyme ADAR2 co-localize in the motor neurons of amyotrophic lateral sclerosis patients, but how they are linked is not clear. Here we demonstrate that activation of calpain, a Ca 2+ -dependent cysteine protease, by upregulation of Ca 2+ -permeable AMPA receptors generates carboxy-terminal-cleaved TDP-43 fragments and causes mislocalization of TDP-43 in the motor neurons expressing glutamine/arginine site-unedited GluA2 of conditional ADAR2 knockout (AR2) mice that mimic the amyotrophic lateral sclerosis pathology. These abnormalities are inhibited in the AR2res mice that express Ca 2+ -impermeable AMPA receptors in the absence of ADAR2 and in the calpastatin transgenic mice, but are exaggerated in the calpastatin knockout mice. Additional demonstration of calpain-dependent TDP43 fragments in the spinal cord and brain of amyotrophic lateral sclerosis patients, and high vulnerability of amyotrophic lateral sclerosis-linked mutant TDP43 to cleavage by calpain support the crucial role of the calpain-dependent cleavage of TDP43 in the amyotrophic lateral sclerosis pathology. Amyotrophic lateral sclerosis (ALS) is the most common adult-onset motor neuron disease affecting healthy middle-aged individuals. The disease course is rapidly progressive, and the eventual respiratory muscle weakness results in death within a few years of onset. The cause of ALS is largely unknown, but transactive response DNA-binding protein 43 (TDP-43), a nuclear protein involved in the regulation of RNA processing [1] , [2] , [3] , [4] , [5] , [6] , [7] , has recently attracted interest as a molecule relevant to the pathogenesis of this disease. TDP-43 is absent from the nucleus in which it normally resides but localizes in abnormal cytoplasmic inclusions in a considerable proportion of spinal cord motor neurons in the majority of sporadic ALS patients [8] , [9] , [10] . As TDP-43 is indispensable for embryonic development and neuronal cell survival in cell culture [2] , [3] , [4] , [7] and genetically modified animals [1] , abnormal localization of TDP-43 in ALS motor neurons is believed to have a pathogenic role in ALS. Molecular abnormalities specifically occurring in motor neurons of patients with sporadic ALS other than TDP-43 pathology include the expression of glutamine/arginine (Q/R) site-unedited GluA2, a subunit of α-amino-3-hydroxy-5-methylisoxazole-4-propionic acid (AMPA) receptors [11] , [12] . This molecular abnormality specifically results from reduced levels of an RNA-editing enzyme called adenosine deaminase acting on RNA 2 (ADAR2) among other members of the ADAR family [13] , [14] . ADAR2 specifically catalyses adenosine (A) to inosine (I; A-to-I) conversion [15] at the Q/R site of GluA2 pre-mRNA [16] , thereby making AMPA receptors impermeable to Ca 2+ (ref. 17 ). ADAR2 activity at the GluA2 Q/R site is indispensable for motor neuron survival, because motor neurons lacking ADAR2 undergo slow death specifically via a failure of GluA2 RNA editing, which results in the upregulation of Ca 2+ -permeable AMPA receptors [18] . Notably, motor neurons devoid of ADAR2 immunoreactivity exhibited TDP-43 pathology and those with ADAR2 immunoreactivity exhibited normal TDP-43 immunoreactivity in ALS patients [13] . The close association of TDP-43 pathology with ADAR2 downregulation suggests a molecular link between the two molecular abnormalities. Owing to the crucial roles of TDP-43 and ADAR2 in neuronal death and their specificity to ALS motor neurons, elucidation of the molecular mechanisms of how they are linked will be indispensable for understanding ALS pathogenesis. We have recently reported that alteration of wild-type and ALS-linked mutant TDP-43 does not affect the level of ADAR2 in cultured cells [19] , indicating that TDP-43 pathology is not the cause of ADAR2 downregulation. Therefore, it is necessary to test whether the downregulation of ADAR2 is critical for generating TDP-43 pathology. Abnormal TDP-43 fragments are present in the central nervous system (CNS) of patients with ALS and frontotemporal lobar degeneration with TDP-43-positive inclusions (FTLD-TDP) [9] , [20] and it is believed that abnormally cleaved, aggregation-prone TDP-43 fragments serve as seeds for cytoplasmic inclusions and that normal, nuclear TDP-43 is sequestered by these inclusions when it shuttles between the nucleus and the cytoplasm [21] . However, the mechanism by which TDP-43 is cleaved into aggregation-prone fragments is unknown. Although the caspase-dependent proteolysis of the TDP-43 amino terminus generates abnormal C-terminal fragments (CTFs) [3] , [4] , [10] , [20] , [22] , the presence of caspase-independent TDP-43 CTFs in the urea fraction of FTLD brain extracts [4] and in a caspase-3 −/− cell line [23] suggests that undetermined proteases also have a significant role in TDP-43 cleavage in the neurons exhibiting TDP-43 pathology. As the downregulation of ADAR2 results in the upregulation of Ca 2+ -permeable AMPA receptors, investigation into a role for Ca 2+ -dependent proteases in the generation of TDP-43 pathology is necessary. Here we report evidence demonstrating that Ca 2+ -dependent cysteine protease calpains cleave the C terminus of TDP-43 and have a crucial role in generating TDP-43 pathology in the motor neurons of ALS model systems and human tissues. As TDP-43 pathology is observed in motor neurons of patients with ALS associated with mutations of the gene encoding TDP-43 ( TARDBP ) and those with sporadic ALS [24] , we also present different hypothetical mechanisms for the generation of aggregation-prone, calpain-dependent TDP-43 fragments in TARDBP -associated ALS and sporadic ALS. Sporadic ALS model mice exhibit TDP-43 pathology To test whether ADAR2 downregulation causes TDP-43 pathology, we examined the subcellular localization of TDP-43 in motor neurons of ADAR2 flox/flox /VAChT-Cre.Fast (AR2) mice in which the gene encoding ADAR2 is conditionally targeted in motor neurons [18] . Approximately half of the motor neurons were devoid of ADAR2 activity and expressed only Q/R site-unedited GluA2, AR2 mice exhibited motor dysfunctions as a result of the slow death of ADAR2-lacking motor neurons [18] . Spinal cord motor neurons lacking ADAR2 were devoid of TDP-43 immunoreactivity in both the nucleus and the cytoplasm, whereas neurons that expressed ADAR2 had TDP-43-positive nuclei, similar to the motor neurons in control mice ( Fig. 1a and Supplementary Fig. S1 ). The spinal cords of AR2 mice showed robust activation of calpain-I and decreased levels of full-length TDP-43 ( Fig. 1b ). We also observed a slight increase in the levels of activated caspase-3 and calpain- and caspase-dependent α-spectrin breakdown products in AR2 mice ( Fig. 1b ). Notably, TDP-43 fragments with molecular masses similar to those observed in the lysates of Neuro2a cells treated with calpain-I were observed in the spinal cord of AR2 mice ( Fig. 1c , arrowheads). 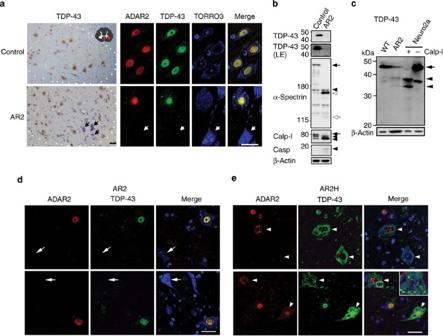Figure 1: TDP-43 mislocalization in the motor neurons of AR2 mice. (a) Immunohistochemistry for TDP-43 demonstrated that TDP-43 localized to the nucleus in all of the large anterior horn cells (AHCs) in control mice, whereas some AHCs in AR2 mice were devoid of TDP-43 expression (arrows). Sections were counterstained with hematoxylin. Immunofluorescence assays revealed that ADAR2 (red) and TDP-43 (green) both localize to the nucleus in control AHCs, but the AR2 AHCs that lack nuclear TDP-43 immunoreactivity are also devoid of ADAR2 immunoreactivity (see the quantification data inSupplementary Fig. S1). TO-PRO-3 (blue) was used as a cell marker. Scale bars, 20 μm. (b) There was a marked decrease in full-length TDP-43 in the spinal cord lysates of AR2 mice compared with wild-type littermates. Consistent with a marked reduction of α-spectrin (black arrow) in association with the generation of calpain- (black and white arrowhead) and caspase-dependent (white arrow and black arrowheads) α-spectrin breakdown products, levels of active calpain-I and caspase-3 (arrowheads) are increased in the AR2 mouse. Arrow, inactive calpain; LE, long exposure. (c) The ~35-kDa bands in the AR2 mice spinal cord correspond to calpain-I-dependent TDP-43 products (arrowheads) in the lysates of Neuro2a cells treated with calpain-I (Calp-I). The samples of AR2 mice spinal cord were loading of gel with five volumes of wild type. Arrow: full-length TDP-43. (d) TDP-43 immunoreactivity was absent in AHCs that lack ADAR2 (arrows) in AR2 mice at 7 weeks and 26 weeks of age. (e) AHCs with low immunoreactivity for ADAR2 (arrowheads) showed TDP-43 immunoreactivity in the cytoplasm in heterozygous AR2 (AR2H) mice at 17 weeks of age. TDP-43-positive cytoplasmic aggregates were seen as well (inset). Figure 1: TDP-43 mislocalization in the motor neurons of AR2 mice. ( a ) Immunohistochemistry for TDP-43 demonstrated that TDP-43 localized to the nucleus in all of the large anterior horn cells (AHCs) in control mice, whereas some AHCs in AR2 mice were devoid of TDP-43 expression (arrows). Sections were counterstained with hematoxylin. Immunofluorescence assays revealed that ADAR2 (red) and TDP-43 (green) both localize to the nucleus in control AHCs, but the AR2 AHCs that lack nuclear TDP-43 immunoreactivity are also devoid of ADAR2 immunoreactivity (see the quantification data in Supplementary Fig. S1 ). TO-PRO-3 (blue) was used as a cell marker. Scale bars, 20 μm. ( b ) There was a marked decrease in full-length TDP-43 in the spinal cord lysates of AR2 mice compared with wild-type littermates. Consistent with a marked reduction of α-spectrin (black arrow) in association with the generation of calpain- (black and white arrowhead) and caspase-dependent (white arrow and black arrowheads) α-spectrin breakdown products, levels of active calpain-I and caspase-3 (arrowheads) are increased in the AR2 mouse. Arrow, inactive calpain; LE, long exposure. ( c ) The ~35-kDa bands in the AR2 mice spinal cord correspond to calpain-I-dependent TDP-43 products (arrowheads) in the lysates of Neuro2a cells treated with calpain-I (Calp-I). The samples of AR2 mice spinal cord were loading of gel with five volumes of wild type. Arrow: full-length TDP-43. ( d ) TDP-43 immunoreactivity was absent in AHCs that lack ADAR2 (arrows) in AR2 mice at 7 weeks and 26 weeks of age. ( e ) AHCs with low immunoreactivity for ADAR2 (arrowheads) showed TDP-43 immunoreactivity in the cytoplasm in heterozygous AR2 (AR2H) mice at 17 weeks of age. TDP-43-positive cytoplasmic aggregates were seen as well (inset). Full size image When changes in the localization of TDP-43 were compared between AR2 mice and heterozygous AR2 mice (AR2H mice; ADAR2 flox/+ /VAChT-Cre.Fast) [25] in which only one ADAR2 allele was targeted, the motor neurons lacking nuclear ADAR2 immunoreactivity were already devoid of nuclear and cytoplasmic TDP-43 immunoreactivity in 7-week-old homozygous AR2 mice ( Fig. 1d , arrows), whereas some motor neurons with low levels of ADAR2 showed TDP-43 immunoreactivity in the cytoplasm with several small TDP-43-positive cytoplasmic aggregates in AR2H mice at 17 weeks of age ( Fig. 1e , arrowheads). The extent of expression of TDP-43 mRNA did not significantly change in AR2, AR2H or wild-type mice at 12 weeks age ( Supplementary Fig. S2 ). Calpains in the spinal cord were markedly upregulated in AR2 mice and slightly upregulated in AR2H mice ( Supplementary Figs S3 and S4 ). As motor neurons with one ADAR2 allele expressed unedited GluA2 to the extent of not >30% of the total GluA2 mRNA in AR2H mice [25] , we concluded that mislocalization of TDP-43 occurs in response to the calpain activation that is associated with ADAR2 downregulation in AR2 and AR2H mice and that the severity of the pathology depends on the level of Q/R site-unedited GluA2. Calpain specifically cleaves TDP-43 We next investigated whether calpain specifically cleaves TDP-43 in cultured cells. Treatment of Neuro2a cell lysates with 0.5 units of calpain-I generated three major fragments of TDP-43 with approximate molecular masses of 33, 34 and 36 kDa ( Fig. 2a ). In contrast, cleavage of TDP-43 was virtually absent in the same lysates treated with 3.0 units of caspase-3, an amount that effectively cleaves α-spectrin ( Fig. 2a ). To confirm that calpain specifically cleaves TDP-43, we performed an in vitro calpain cleavage assay using recombinant human TDP-43 and Neuro2a cell lysates. The amount of full-length human and mouse TDP-43 decreased in a time- and concentration-dependent manner in the presence of calpain-I or calpain-II ( Fig. 2b–d ). Calpain-dependent TDP-43 cleavage was effectively inhibited in the presence of specific calpain inhibitors (MDL28170 and ALLN) or the general cysteine protease inhibitor leupeptin but not in the presence of the caspase inhibitor Z-VAD-FMK or the CDK5 inhibitor roscovitine ( Fig. 2e ). Therefore, calpain specifically cleaves human and mouse TDP-43. 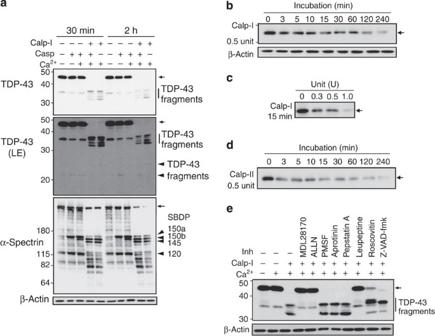Figure 2: Calpain-dependent cleavage of TDP-43in vitro. (a) Neuro2a cell lysates were analysed by western blotting with TDP-43 antibodies after treatment with calpain-I (Calp-I), caspase-3 (Casp) and/or CaCl2(Ca2+). Calpain cleaved TDP-43 into fragments with an apparent molecular mass of 33–36 kDa, whereas caspase-3 failed to cleave TDP-43 at the concentration that effectively cleaved α-spectrin. The activation of calpain and caspase-3 was demonstrated by the cleavage of α-spectrin into calpain-dependent spectrin breakdown products (SBDP) (150b and 145) and caspase-3-dependent SBDP (150a and 120). (b,c) Levels of recombinant human TDP-43 declined in the presence of calpain-I in a time-dependent (b) and a concentration-dependent manner (c). (d) Calpain-II cleaved recombinant human TDP-43 in the same manner as calpain-I. (e) Inhibitors (inh) of calpain (MDL28170, ALLN and leupeptin) but not inh of other proteases (phenylmethylsulphonyl fluoride (PMSF), aprotinin, pepstatin, roscovitine and Z-VAD-fmk) effectively inhibited the calpain-dependent cleavage of TDP-43 in Neuro2a cell lysates. Arrows, full-length proteins. Figure 2: Calpain-dependent cleavage of TDP-43 in vitro . ( a ) Neuro2a cell lysates were analysed by western blotting with TDP-43 antibodies after treatment with calpain-I (Calp-I), caspase-3 (Casp) and/or CaCl 2 (Ca 2+ ). Calpain cleaved TDP-43 into fragments with an apparent molecular mass of 33–36 kDa, whereas caspase-3 failed to cleave TDP-43 at the concentration that effectively cleaved α-spectrin. The activation of calpain and caspase-3 was demonstrated by the cleavage of α-spectrin into calpain-dependent spectrin breakdown products (SBDP) (150b and 145) and caspase-3-dependent SBDP (150a and 120). ( b , c ) Levels of recombinant human TDP-43 declined in the presence of calpain-I in a time-dependent ( b ) and a concentration-dependent manner ( c ). ( d ) Calpain-II cleaved recombinant human TDP-43 in the same manner as calpain-I. ( e ) Inhibitors (inh) of calpain (MDL28170, ALLN and leupeptin) but not inh of other proteases (phenylmethylsulphonyl fluoride (PMSF), aprotinin, pepstatin, roscovitine and Z-VAD-fmk) effectively inhibited the calpain-dependent cleavage of TDP-43 in Neuro2a cell lysates. Arrows, full-length proteins. Full size image Cleavage and mislocalization of TDP-43 are calpain dependent To test whether the mislocalization of TDP-43 in AR2 mice was induced by activation of calpain in response to amplified Ca 2+ influx through AMPA receptors, we investigated changes in TDP-43 and calpains in AR2res (AR2/GluR- B R/R ) mice [18] . In these mice, the endogenous GluA2 alleles have been replaced with the GluR-B R allele, which encodes a Q/R site-edited GluA2. Mutant neurons therefore express Ca 2+ -impermeable AMPA receptors with edited GluA2, even in the absence of ADAR2 (ref. 26 ). Neither the abnormal TDP-43 fragments ( Fig. 3a ) nor activated calpains were detected in AR2res mice at 6 months of age ( Fig. 3a and Supplementary Fig. S3b –d). Moreover, motor neurons lacking ADAR2 immunoreactivity displayed normal TDP-43 immunoreactivity in AR2res mice at 6 months of age ( Fig. 3c , arrows). In addition, to test whether calpain specifically has a role in the fragmentation and mislocalization of TDP-43 in the mouse brain and spinal cord, we investigated the calpain-dependent cleavage of TDP-43 in the lysates of the brain and spinal cord of knockout (CAST KO) [27] or transgenic (Tg) (CAST Tg) mice [28] for calpastatin (CAST), the endogenous calpain inhitibor. TDP-43 cleavage was accelerated in the absence of CAST and inhibited by the overexpression of CAST ( Fig. 3d ). Activities of both calpain-I and calpain-II were increased in the spinal cords of CAST KO mice compared with control and CAST Tg mice ( Supplementary Fig. S5 ). In accordance with the accelerated cleavage of TDP-43, TDP-43 mislocalized in the cytoplasm in the spinal cord motor neurons of the CAST KO mice ( Fig. 3e ). These data further support the idea that calpain activation via exaggerated Ca 2+ influx through AMPA receptors causes TDP-43 pathology in mouse motor neurons. 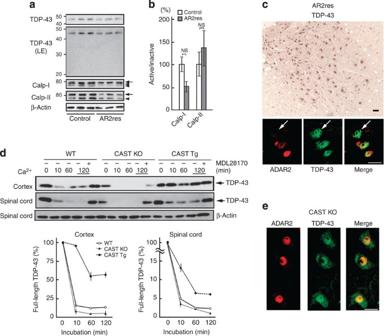Figure 3: Rescue of abnormal calpain-dependent cleavage of TDP-43 in AR2 mice. (a) Immunoblot analyses of spinal cord extracts detected neither abnormal TDP-43 fragments nor an increase in activated forms of calpain in the AR2res mice compared with control mice. (b) Levels of the activated forms of calpain-I and II were not different between AR2res and control mice. The results are presented as the ratio to the value from the control mice shown inSupplementary Fig. S3. Means (columns) and s.e.m. (bars) are indicated (n=3; Student’st-test against the wild-type (WT) value). (c) Immunohistochemical analysis for TDP-43 demonstrated that all AHCs in the AR2res mouse express nuclear TDP-43. Sections were counterstained with hematoxylin. There was normal nuclear TDP-43 immunoreactivity in ADAR2-deficient AHCs (arrow) in the AR2res mouse. (d) Cleavage of TDP-43 by calpain in the brain and spinal cord extracts of Tg (CAST Tg) or knockout (CAST KO) mice for CAST, the endogenous calpain inhibitor protein. Immunoblots show the effects of treatment of the mouse brain or spinal cord extracts with 5 mM Ca2+for the indicated period of time in the presence or absence of 20 mM MDL28170 (calpain inhibitor). The amount of full-length TDP-43 at each time point is expressed as the percentage of that at time 0. Means (symbols) and s.e.m. (bars) are indicated (n=3). (e) Immunohistochemistry for TDP-43 demonstrates that all AHCs express abnormal cytoplasmic TDP-43 immunoreactivity in the CAST KO mouse. Scale bars, 20 μm. Figure 3: Rescue of abnormal calpain-dependent cleavage of TDP-43 in AR2 mice. ( a ) Immunoblot analyses of spinal cord extracts detected neither abnormal TDP-43 fragments nor an increase in activated forms of calpain in the AR2res mice compared with control mice. ( b ) Levels of the activated forms of calpain-I and II were not different between AR2res and control mice. The results are presented as the ratio to the value from the control mice shown in Supplementary Fig. S3 . Means (columns) and s.e.m. (bars) are indicated ( n =3; Student’s t -test against the wild-type (WT) value). ( c ) Immunohistochemical analysis for TDP-43 demonstrated that all AHCs in the AR2res mouse express nuclear TDP-43. Sections were counterstained with hematoxylin. There was normal nuclear TDP-43 immunoreactivity in ADAR2-deficient AHCs (arrow) in the AR2res mouse. ( d ) Cleavage of TDP-43 by calpain in the brain and spinal cord extracts of Tg (CAST Tg) or knockout (CAST KO) mice for CAST, the endogenous calpain inhibitor protein. Immunoblots show the effects of treatment of the mouse brain or spinal cord extracts with 5 mM Ca 2+ for the indicated period of time in the presence or absence of 20 mM MDL28170 (calpain inhibitor). The amount of full-length TDP-43 at each time point is expressed as the percentage of that at time 0. Means (symbols) and s.e.m. (bars) are indicated (n=3). ( e ) Immunohistochemistry for TDP-43 demonstrates that all AHCs express abnormal cytoplasmic TDP-43 immunoreactivity in the CAST KO mouse. Scale bars, 20 μm. Full size image Calpain cleaves the C terminus of TDP-43 We then analysed calpain cleavage sites in TDP-43 using human TDP-43 fused to green fluorescent protein (GFP) at the N terminus (GFP-TDP-43). Calpain treatment of lysates from HeLa cells expressing GFP-TDP-43 generated calpain-dependent fragments of GFP-TDP-43 that were consistently detected with both GFP antibodies and TDP-43 antibodies but not C-terminal-specific TDP-43 antibodies (TDP-43C; epitope: 350-C terminus of human TDP-43; Fig. 4a ). To precisely map the calpain cleavage sites, we performed in vitro calpain cleavage reactions using recombinant HIS 6 -TDP-43 followed by mass spectrometric analysis of the purified calpain-dependent cleavage products ( Fig. 4b ). Treatment of recombinant HIS 6 -TDP-43 with calpain generated three major fragments (band-a to band-c in Fig. 4b ), which corresponded to the calpain-dependent TDP-43 fragments with approximate molecular masses of 36, 34 and 33 kDa ( Fig. 2a ). Each band was excised and digested with trypsin, and the resultant peptides were subjected to matrix-assisted laser desorption/ionization-time of flight mass spectrometry (MALDI-TOF-MS). MS/MS analysis identified 12 peptides in the calpain-dependent fragments (3 peptides in band-c, 4 peptides in band-b from recombinant HIS 6 -TDP-43 and 5 peptides in band-a from recombinant HIS 6 -TDP-43 I318R; Fig. 4c , Supplementary Figs S6–8 and Supplementary Table S1 ). As there was no trypsin site (arginine/lysine) in the vicinity of the putative calpain site for band-a from HIS 6 -TDP-43 ( Fig. 4b , lane 1 band-a), we inserted a mutation at residue 318 (HIS 6 -TDP-43 I318R) in the vicinity of the putative calpain site that generates the 36-kDa fragment of TDP-43. The results indicate that TDP-43 has multiple calpain cleavage sites in the C terminus between amino-acid residues 229 and 346 ( Fig. 4c , Supplementary Fig. S9 and Supplementary Table S1 ). 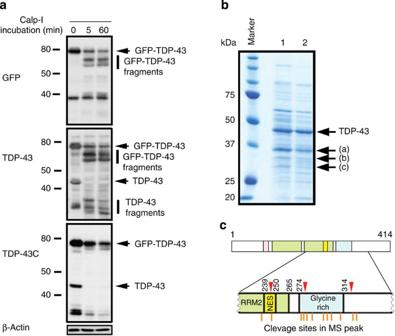Figure 4: Calpain-dependent cleavage of TDP-43 at the C terminus. (a) Western blot analysis of calpain-I-treated HeLa cells transfected with human TDP-43 tagged with GFP at the N terminus (GFP-TDP-43). Fragments of GFP-TDP-43 were recognized with anti-GFP and anti-TDP-43 antibodies but not with antibodies specific to the C terminus of TDP-43 (TDP-43C). (b) Calpain-dependent fragments of recombinant His6-TDP-43 (lane 1) and His6-TDP-43 I318R (lane 2). Full-length TDP-43 and the three major calpain-dependent fragments (a–c) are indicated with arrows. Each of the cleaved TDP-43 products were subjected to MALDI-TOF-MS (seeSupplementary Table S1andSupplementary Figs S6–8). (c) Schematic illustration of the putative calpain cleavage sites in TDP-43 predicted by MALDI-TOF-MS analysis (red arrowheads). Cleavage sites of peptides corresponding to the mass peaks detected are mapped on the primary sequence of TDP-43 (orange bars; between amino acids 229 and 346). The details are also summarized inSupplementary Table S1. Figure 4: Calpain-dependent cleavage of TDP-43 at the C terminus. ( a ) Western blot analysis of calpain-I-treated HeLa cells transfected with human TDP-43 tagged with GFP at the N terminus (GFP-TDP-43). Fragments of GFP-TDP-43 were recognized with anti-GFP and anti-TDP-43 antibodies but not with antibodies specific to the C terminus of TDP-43 (TDP-43C). ( b ) Calpain-dependent fragments of recombinant His 6 -TDP-43 (lane 1) and His 6 -TDP-43 I318R (lane 2). Full-length TDP-43 and the three major calpain-dependent fragments ( a – c ) are indicated with arrows. Each of the cleaved TDP-43 products were subjected to MALDI-TOF-MS (see Supplementary Table S1 and Supplementary Figs S6–8 ). ( c ) Schematic illustration of the putative calpain cleavage sites in TDP-43 predicted by MALDI-TOF-MS analysis (red arrowheads). Cleavage sites of peptides corresponding to the mass peaks detected are mapped on the primary sequence of TDP-43 (orange bars; between amino acids 229 and 346). The details are also summarized in Supplementary Table S1 . Full size image We next investigated whether the calpain-dependent TDP-43 fragments had aggregation-prone properties in HeLa cells using GFP-tagged TDP-43 fragments ( Fig. 5a ). Transfection with large calpain-dependent TDP-43 fragments (1–286 and 1–324) induced larger cytoplasmic aggregates in a significantly higher proportion of cells as compared with the transfection of full-length TDP-43, whereas transfection of the small fragment (1–243) induced small aggregates with diffuse TDP-43 staining, similar to the transfection of full-length TDP-43 ( Fig. 5b ). Next, we tested the role of the calpain-dependent CTFs of TDP-43 using human TDP-43 fused with GFP at the C terminus (TDP-43-GFP). We found that the calpain-dependent TDP-43-GFP fragments had approximate molecular masses of 37 and 34 kDa by immunoblotting for GFP ( Supplementary Fig. S10a ), indicating that the CTFs have molecular masses of 10 kDa or less. In addition, the GFP-tagged CTFs (324–414; Supplementary Fig. S10b ) had no aggregation-prone properties in cultured cells ( Supplementary Fig. S10c ), although the relatively large and soluble GFP protein may have affected the solubility of the small TDP-43 fragments. These results indicate that calpain serially cleaves TDP-43 into aggregation-prone large fragments and further into smaller fragments that are no longer aggregation-prone ( Fig. 5d ). 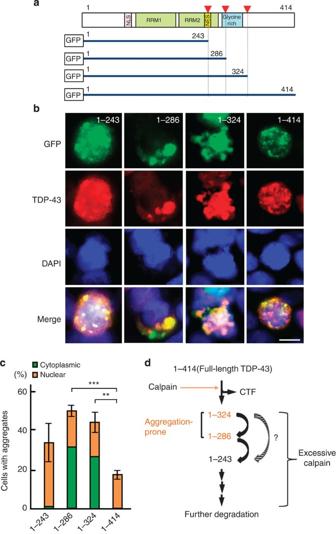Figure 5: Aggregation of calpain-dependent TDP-43 fragments. (a) The three main calpain-cleaved sites of TDP-43 (red arrowheads) and the calpain-dependent TDP-43 fragment constructs tagged with GFP at the N terminus are illustrated. (b) Examples of cells 72 h after transfection with the GFP-TDP-43 fragment or with GFP-TDP-43. The numbers in the rows indicate the constructs indicated ina. The cells transfected with the constructs of larger calpain-dependent TDP-43 fragments (1–286, 1–324) exhibited large and extensive aggregates, whereas those transfected with the constructs of the full-length TDP-43 or the small calpain-dependent TDP-43 fragment (1–243) exhibited small aggregates with diffuse TDP-43 immunoreactivity. The nuclei were visualized with 4,6-diamidino-2-phenylindole (DAPI). Scale bar, 10 μm. (c) The proportion of cells with aggregates among those exhibiting GFP signals was calculated. The larger calpain-dependent TDP-43 fragments (1–286 and 1–324) induced cytoplasmic aggregations in a larger number of cells than the full-length TDP-43 or the small calpain-dependent TDP-43 fragment (1–243). Means (columns) and s.e.m. (bars) are indicated (n=3; ***P=0.0036; and **P=0.0115, Student’st-test against the wild-type value). (d) Schematic illustration of sequential cleavage of TDP-43 by calpain. Activation of calpain generates aggregation-prone N-terminal fragments (orange), which are sequentially cleaved into smaller fragments that are no longer aggregation-prone. CTFs of TDP-43 are not prone to aggregation. Figure 5: Aggregation of calpain-dependent TDP-43 fragments. ( a ) The three main calpain-cleaved sites of TDP-43 (red arrowheads) and the calpain-dependent TDP-43 fragment constructs tagged with GFP at the N terminus are illustrated. ( b ) Examples of cells 72 h after transfection with the GFP-TDP-43 fragment or with GFP-TDP-43. The numbers in the rows indicate the constructs indicated in a . The cells transfected with the constructs of larger calpain-dependent TDP-43 fragments (1–286, 1–324) exhibited large and extensive aggregates, whereas those transfected with the constructs of the full-length TDP-43 or the small calpain-dependent TDP-43 fragment (1–243) exhibited small aggregates with diffuse TDP-43 immunoreactivity. The nuclei were visualized with 4,6-diamidino-2-phenylindole (DAPI). Scale bar, 10 μm. ( c ) The proportion of cells with aggregates among those exhibiting GFP signals was calculated. The larger calpain-dependent TDP-43 fragments (1–286 and 1–324) induced cytoplasmic aggregations in a larger number of cells than the full-length TDP-43 or the small calpain-dependent TDP-43 fragment (1–243). Means (columns) and s.e.m. (bars) are indicated ( n =3; *** P =0.0036; and ** P =0.0115, Student’s t -test against the wild-type value). ( d ) Schematic illustration of sequential cleavage of TDP-43 by calpain. Activation of calpain generates aggregation-prone N-terminal fragments (orange), which are sequentially cleaved into smaller fragments that are no longer aggregation-prone. CTFs of TDP-43 are not prone to aggregation. Full size image Activated calpain cleaves TDP-43 in ALS patients Next, using general TDP-43 antibodies and TDP-43C, we examined whether the calpain-dependent TDP-43 fragments lacking the C terminus were expressed in the CNS of affected patients. When the specificity of the TDP-43C antibodies was tested in HeLa cell lysates, they failed to recognize all of the calpain-dependent fragments that were recognized by general TDP-43 antibodies ( Supplementary Fig. S11 , lanes 2–6), indicating that TDP-43C antibodies detected caspase-3-dependent TDP-43 CTFs but not calpain-dependent N-terminal fragments of TDP-43 ( Supplementary Fig. S11 , lane 7). In the spinal cords and primary motor cortices of patients with ALS with dementia (FTLD-motor neuron disease; (FTLD-MND)) in which pathological 25- to 28-kDa TDP-43 fragments were detected, there was an increase in the levels of activated calpain-I and calpain-II compared with the control subjects ( Fig. 6a–d and Supplementary Fig. S12 ). The TDP-43C antibodies did not recognize abnormal fragments in the CNS lysates ( Supplementary Fig. S12 ) and faintly recognized the 25- to 28-kDa fragments but did not recognize the 35-kDa bands that were identified with antibodies against full-length TDP-43 and phosphorylated TDP-43 (TDP-43pS409/410) in urea-soluble fractions ( Fig. 6e ). These results suggest that some of the abnormal TDP-43 fragments in ALS CNS tissue lack the C-terminal end and are generated by calpain cleavage. Consistent with previous reports on cultured human cells treated with staurosporine [20] , [29] , treatment of HeLa cell lysates with a large amount (ten units) of caspase-3 generated fragments with an apparent molecular mass of 35-kDa ( Fig. 6f , open asterisk). Notably, sequential treatment of HeLa cell lysates with calpain- and caspase-3-generated fragments that corresponded to the abnormal 25- to 28-kDa TDP-43 fragments observed in the urea-soluble brain extracts from patients ( Fig. 6f , filled asterisk). These results suggest that calpain and caspase-3 act in concert to cleave human TDP-43 into the corresponding pathological fragments. 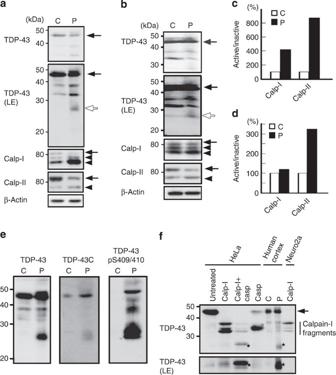Figure 6: Roles of calpain (Calp) in TDP-43 pathology in ALS. (a,b) Immunoblot analyses of total homogenates from the primary motor cortex of an FTLD-MND patient (a) and the spinal cord of an ALS patient (b). Abnormal TDP-43 fragments (white arrow) were present in patient tissues (P) in association with increased levels of activated Calp-I and Calp-II (arrowheads) relative to control tissues (C) (seeSupplementary Fig. S12). Black arrows indicate full-length TDP-43 and inactive Calp-I and Calp-II. β-Actin was used as a loading control. LE, long exposure. (c,d) Densitometric quantification of the relative intensity of the bands ina(c) andb(d) revealed a marked increase of activated Calps relative to inactive forms in the patient tissues (filled columns) compared with the control tissues (open columns). (e) Abnormal TDP-43 fragments in the brain of an FTLD-MND patient (P). The C-terminal-specific TDP-43 antibodies (TDP-43C) did not recognize the ~35-kDa bands and only faintly recognized the ~25-kDa bands that were recognized by the antibodies against total TDP-43 and phosphorylated TDP-43 (TDP-43pS409/410) in the sarkosyl-insoluble fraction. (f) Bands of the ~25-kDa TDP-43 fragments corresponding to those in the sarkosyl-insoluble fraction of the FTLD-MND brain (filled asterisk) were only observed in the lysates of HeLa cells treated concomitantly with Calp-I and caspase-3 (Casp). The ~35-kDa bands in the FTLD-MND brain correspond to Calp-I-dependent TDP-43 products but not to Casp-dependent products (open asterisk) in the HeLa cell lysates. Figure 6: Roles of calpain (Calp) in TDP-43 pathology in ALS. ( a , b ) Immunoblot analyses of total homogenates from the primary motor cortex of an FTLD-MND patient ( a ) and the spinal cord of an ALS patient ( b ). Abnormal TDP-43 fragments (white arrow) were present in patient tissues (P) in association with increased levels of activated Calp-I and Calp-II (arrowheads) relative to control tissues (C) (see Supplementary Fig. S12 ). Black arrows indicate full-length TDP-43 and inactive Calp-I and Calp-II. β-Actin was used as a loading control. LE, long exposure. ( c , d ) Densitometric quantification of the relative intensity of the bands in a ( c ) and b ( d ) revealed a marked increase of activated Calps relative to inactive forms in the patient tissues (filled columns) compared with the control tissues (open columns). ( e ) Abnormal TDP-43 fragments in the brain of an FTLD-MND patient (P). The C-terminal-specific TDP-43 antibodies (TDP-43C) did not recognize the ~35-kDa bands and only faintly recognized the ~25-kDa bands that were recognized by the antibodies against total TDP-43 and phosphorylated TDP-43 (TDP-43pS409/410) in the sarkosyl-insoluble fraction. ( f ) Bands of the ~25-kDa TDP-43 fragments corresponding to those in the sarkosyl-insoluble fraction of the FTLD-MND brain (filled asterisk) were only observed in the lysates of HeLa cells treated concomitantly with Calp-I and caspase-3 (Casp). The ~35-kDa bands in the FTLD-MND brain correspond to Calp-I-dependent TDP-43 products but not to Casp-dependent products (open asterisk) in the HeLa cell lysates. Full size image ALS-linked mutant TDP-43 is highly vulnerable to clapain As most of the ALS-linked point mutations in the TARDBP gene are localized to the C terminus [30] , [31] , we investigated the kinetic differences between the calpain-dependent cleavage of ALS-linked mutant TDP-43 and wild-type TDP-43. We found that calpain-I digested recombinant ALS-linked TDP-43 A315T and TDP-43 M337V faster than wild-type TDP-43 in vitro ( Fig. 7a ). When regional differences in calpain activity were investigated in normal human brains and spinal cords, activated calpain and calpain-dependent TDP-43 fragments were more abundantly expressed in the ventral grey matter of the spinal cord than in the dorsal grey matter or primary motor cortex ( Fig. 7c ,d). 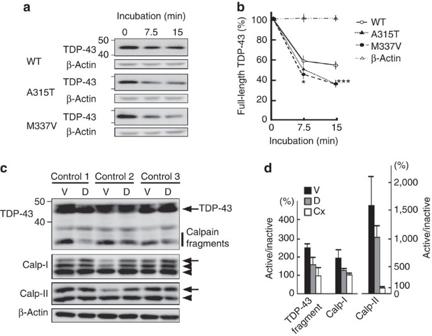Figure 7: Roles of calpain inTARDBP-associated ALS. (a) Calpain-dependent cleavage of ALS-linked mutant TDP-43. Calpain-I cleaved TDP-43A315T(A315T) and TDP-43M337V(M337V) more efficiently than wild-type TDP-43 (WT). (b) The amount of full-length TDP-43 at each time point inais expressed as the percentage of that at time 0. Means (symbols) and s.e.m. (bars) are indicated (n=5; *P=0.037; and ***P<0.005, Student’st-test against the WT value). (c) An immunoblot analysis revealed an increase in the levels of calpain-dependent TDP-43 fragments along with an increase of activated calpain-I and calpain-II (arrowheads) in the ventral grey matter (V) of the spinal cord compared with the dorsal grey matter (D). Arrows indicate the full-length proteins. (d) The relative expression levels of calpain-dependent TDP-43 fragments compared with full-length TDP-43 (arrow inc) and those of the activated forms of calpain-I and calpain-II relative to their respective inactive forms (arrows inc) were calculated by quantifying the densitometric intensity of the corresponding bands inc. The results are presented as the ratio relative to the value in the motor cortex (Cx;n=3) shown inSupplementary Fig. S12b. Note that activated calpains and calpain-dependent TDP-43 fragments are most abundant in the ventral grey matter (V) of the spinal cord. The data are presented as the mean (columns) and s.e.m. (bars). β-Actin was used as a loading control. Figure 7: Roles of calpain in TARDBP -associated ALS. ( a ) Calpain-dependent cleavage of ALS-linked mutant TDP-43. Calpain-I cleaved TDP-43 A315T (A315T) and TDP-43 M337V (M337V) more efficiently than wild-type TDP-43 (WT). ( b ) The amount of full-length TDP-43 at each time point in a is expressed as the percentage of that at time 0. Means (symbols) and s.e.m. (bars) are indicated ( n =5; * P =0.037; and *** P <0.005, Student’s t -test against the WT value). ( c ) An immunoblot analysis revealed an increase in the levels of calpain-dependent TDP-43 fragments along with an increase of activated calpain-I and calpain-II (arrowheads) in the ventral grey matter (V) of the spinal cord compared with the dorsal grey matter (D). Arrows indicate the full-length proteins. ( d ) The relative expression levels of calpain-dependent TDP-43 fragments compared with full-length TDP-43 (arrow in c ) and those of the activated forms of calpain-I and calpain-II relative to their respective inactive forms (arrows in c ) were calculated by quantifying the densitometric intensity of the corresponding bands in c . The results are presented as the ratio relative to the value in the motor cortex (Cx; n =3) shown in Supplementary Fig. S12b . Note that activated calpains and calpain-dependent TDP-43 fragments are most abundant in the ventral grey matter (V) of the spinal cord. The data are presented as the mean (columns) and s.e.m. (bars). β-Actin was used as a loading control. Full size image In the present paper, we demonstrated that dying motor neurons in AR2 (ADAR2 flox/flox /VAChT-Cre.Fast) mice expressing Ca 2+ -permeable AMPA receptors exhibited TDP-43 mislocalization that mimics the molecular pathology seen in the motor neurons of sporadic ALS patients. We showed that calpain was activated by the downregulation of ADAR2 and that calpain cleaved TDP-43 in the C-terminal region, inducing the generation of aggregation-prone fragments and the mislocalization of TDP-43. TDP-43 mislocalization was reversed by the normalization of calpain activity in AR2res (AR2/GluR- B R/R ) mice, in which normal Ca 2+ -impermeable AMPA receptors were expressed in the absence of ADAR2. Cleavage of TDP-43 was effectively affected by the activity of the endogenous calpain inhibitor CAST in the brains and spinal cords. Notably, calpain-dependent TDP-43 fragments were present in affected CNS tissues of ALS patients, in which calpain activity was increased. These results suggest that an increase in Ca 2+ influx through the upregulation of Ca 2+ -permeable AMPA receptors containing Q/R site-unedited GluA2 activates calpain and that the exaggerated calpain-dependent cleavage of TDP-43 has a crucial role in TDP-43 pathology in ALS motor neurons. The findings that ADAR2 activity is already reduced in ALS motor neurons before they express unedited GluA2 or exhibit TDP-43 pathology [14] and that ADAR2 activity does not change after the overexpression or knockdown of TDP-43 or the expression of TDP-43 fragments or mutant TDP-43 in cultured cells [19] lend further support to our conclusion that the downregulation of ADAR2 is likely an upstream event in the molecular mechanism of TDP-43 pathology in ALS motor neurons [13] . We observed the disappearance of TDP-43 in AR2 mice in the early postnatal weeks but observed cytoplasmic mislocalization of TDP-43 concurrent with the formation of aggregates in the motor neurons of heterozygous AR2H mice ( Fig. 1d ). ADAR2-lacking motor neurons in AR2 mice express only Q/R site-unedited GluA2, whereas ADAR2-targetted motor neurons in heterozygous AR2H mice express unedited GluA2 mRNA to an extent of <30% of the total GluA2 mRNA [25] . This implies that the expression of Ca 2+ -permeable AMPA receptors and hence the Ca 2+ influx in motor neurons was lower in AR2H mice than in AR2 mice. Indeed, the level of Ca 2+ influx through the AMPA receptors differed according to the expression level of unedited GluA2 in the mutant mice; a 29-fold increase in Ca 2+ influx was observed in mice expressing only unedited GluA2 and a 4.5-fold increase was observed in mice expressing unedited GluA2, representing 45% of the total GluA2 protein compared with wild-type mice that express only edited GluA2 (ref. 32 ). It is therefore likely that different levels of unedited GluA2 result in different levels of active calpain and the resultant cleavage of TDP-43 in our AR2 and AR2H mice. The presence of cytoplasmic aggregates in the AR2H mouse motor neurons suggests the generation of aggregation-prone fragments. TDP-43 possesses a putative prion domain in the C-terminal region that is prone to aggregation [3] , [4] , [6] , [33] , and the aggregation activity is highest in the regions of amino acids 277–400 (ref. 33 ) and 287–322 (ref. 34 ). Among the major calpain-dependent N-terminal fragments of TDP-43, fragments 1–286 and 1–324 were aggregation-prone, but the smallest fragment 1–243, was not. Exaggerated calpain activity cleaved the large fragments 1–286 and 1–324 into the 1–243 or smaller fragments that were no longer aggregation-prone ( Fig. 5 and Supplementary Fig. S13 ). Therefore, the higher calpain activity in the motor neurons of the AR2 mice rapidly cleaved TDP-43 into small non-aggregating fragments, whereas a more modest rise in calpain activity in the motor neurons of the AR2H mice left the aggregation-prone TDP-43 fragments intact. It is likely that extremely high or extremely low calpain activity does not generate TDP-43 pathology, and that a modest increase in Ca 2+ influx through AMPA receptors in conjunction with the modest activation of calpain is suitable for the generation of TDP-43 pathology in motor neurons of ALS patients that express various proportions of unedited GluA2 (refs 12 , 14 ). As normal TDP-43 is highly expressed in the nucleus and at low levels in the cytoplasm shuttling between the nucleus and the cytoplasm [35] , once small aggregates are formed, they may serve as seeds for inclusions that sequester TDP-43, thereby generating large cytoplasmic inclusions. A pathogenic role for TDP-43 CTFs lacking the C-terminal end in ALS is supported by evidence from one ALS patient carrying a Y374X nonsense mutation in the TARDBP gene that generated C-terminal-truncated TDP-43 (ref. 5 ). Various fragments have been identified in the brains and spinal cords of FTLD-TDP and ALS patients [3] , [4] , [8] , [9] , [10] , [20] but the role of N-terminal fragments has not been attracted the attention of researchers. In this study, we show that calpain cleaves the C-terminal region of TDP-43 and generates multiple different fragments by sequentially cleaving the large N-terminal fragments. The presence of TDP-43 CTFs and fragments consistent with those generated by cleavage with both calpain and caspase-3 ( Fig. 6f ) suggests the participation of caspase-3, as previously argued [3] , [20] . Although the calpain-dependent fragments of TDP-43 can serve as seeds for inclusion, the activation of caspase-3 by excitotoxic neuronal damage in mice [27] suggests that caspase-3 may participate in the generation of TDP-43 pathology by cleaving the full-length and calpain-dependent fragments of TDP-43 into aggregation-prone fragments. TDP-43 pathology appears in the motor neurons of patients with ALS associated with mutations in the TARDBP gene as well as sporadic ALS patients who express wild-type TDP-43 (refs 8 , 9 , 10 , 30 , 31 ). The increased vulnerability of mutant TDP-43 to calpain is in agreement with the fact that most ALS-linked point mutations in the TARDBP gene are localized to the C-terminal region [1] , [30] , [31] . In addition, the CTFs of mutant TDP-43 exhibit much faster kinetics of fibril formation than the CTFs of wild-type TDP-43 (ref. 34 ). It is therefore probable that neurons expressing mutant TDP-43 would be more likely to generate TDP-43 pathology than those expressing wild-type TDP-43. As spinal motor neurons express relatively low levels of GluA2, they contain a high proportion of Ca 2+ -permeable AMPA receptors lacking GluA2 (refs 36 , 37 , 38 ). This property may account for the higher calpain activity observed in spinal motor neurons compared with other CNS regions ( Fig. 7c ). The physiologically higher calpain activity in the ventral horns of the spinal cord may explain why mutations in the TARDBP gene cause ALS but not FTLD-TDP in affected patients [8] , [9] , [10] , [30] , [31] . Our studies of mutant TDP-43 imply that the same neuropathological changes may arise from different molecular mechanisms, that is, protease activation and increased vulnerability of the substrate to the protease. Therefore, it may be necessary to perform separate investigations into the molecular mechanisms underlying sporadic and familial cases of this neurological disease. Taken together, our findings suggest that calpain-dependent cleavage of TDP-43 is likely an initial event leading to the TDP-43 pathology seen in ALS. However, underlying mechanisms are different between sporadic ALS and TARDBP -associated ALS: calpain activation through the upregulation of Ca 2+ -permeable AMPA receptors that contain Q/R site-unedited GluA2 is the theoretical mechanism underlying sporadic ALS, whereas a combination of the increased vulnerability of mutant TDP-43 to calpain with resultant generation of highly aggregation-prone fragments in calpain-rich motor neurons is likely to be the mechanism underlying TARDBP -associated ALS ( Fig. 8 ). 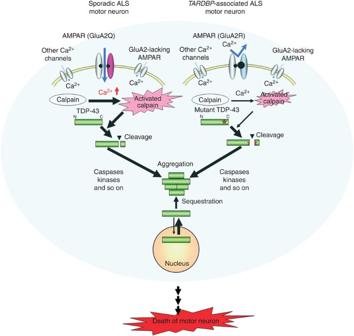Figure 8: Schematic illustration of the molecular mechanisms underlying TDP-43 pathology in ALS motor neurons. Calpain-dependent TDP-43 fragment generation has a crucial role in TDP-43 pathology in both sporadic ALS andTARDBPassociated ALS, but the molecular mechanisms differ. In sporadic ALS, calpain is activated by increased Ca2+influx through the upregulation of Ca2+-permeable AMPA receptors (AMPAR) containing Q/R site-unedited GluA2 (GluA2Q) due to reduced ADAR2 activity. In contrast, the increased vulnerability of mutant TDP-43 to calpain-mediated cleavage generates highly aggregation-prone fragments inTARDBPassociated ALS. Higher levels of activated calpain in the spinal motor neurons relative to the cortex and other brain regions (Fig. 7c,d) may result in the clinical manifestation of ALS rather than FTLD in patients carryingTARDBPmutations. In both sporadic andTARDBPassociated ALS, the aggregation-prone nature of calpain-dependent TDP-43 fragments allows them to serve as seeds for cytoplasmic inclusions. Once an aggregate is generated, TDP-43 proteins shuttling between the nucleus and the cytoplasm may be sequestered in the inclusions, thereby leading to the death of motor neurons via an as yet undefined cascade. Figure 8: Schematic illustration of the molecular mechanisms underlying TDP-43 pathology in ALS motor neurons. Calpain-dependent TDP-43 fragment generation has a crucial role in TDP-43 pathology in both sporadic ALS and TARDBP associated ALS, but the molecular mechanisms differ. In sporadic ALS, calpain is activated by increased Ca 2+ influx through the upregulation of Ca 2+ -permeable AMPA receptors (AMPAR) containing Q/R site-unedited GluA2 (GluA2Q) due to reduced ADAR2 activity. In contrast, the increased vulnerability of mutant TDP-43 to calpain-mediated cleavage generates highly aggregation-prone fragments in TARDBP associated ALS. Higher levels of activated calpain in the spinal motor neurons relative to the cortex and other brain regions ( Fig. 7c ,d) may result in the clinical manifestation of ALS rather than FTLD in patients carrying TARDBP mutations. In both sporadic and TARDBP associated ALS, the aggregation-prone nature of calpain-dependent TDP-43 fragments allows them to serve as seeds for cytoplasmic inclusions. Once an aggregate is generated, TDP-43 proteins shuttling between the nucleus and the cytoplasm may be sequestered in the inclusions, thereby leading to the death of motor neurons via an as yet undefined cascade. Full size image TDP-43 pathology is not specific to ALS motor neurons and FTLD-TDP cortical neurons. It is also observed in various neurological diseases, including Alzheimer’s disease [39] and traumatic brain injury [40] , and in the CNS of animals exposed to various adverse conditions, including sciatic axotomies [41] and brain ischaemia [42] . In addition, mislocalization of TDP-43 from the nucleus to the cytoplasm is observed in the cortical neurons of normal elderly people [43] and motor neurons of aged mice [44] . As a pathogenic role for abnormal Ca 2+ signalling has been proposed in these conditions [36] , [45] , it is likely that activation of Ca 2+ -dependent calpain has a role in the TDP-43 pathology observed in these conditions as well. In addition to Ca 2+ -permeable AMPA receptors, there are multiple sources of intracellular Ca 2+ , including Ca 2+ -permeable receptors and channels, as well as Ca 2+ storage vesicles such as the mitochondria and the endoplasmic reticulum [46] , and Ca 2+ sources responsible for activation of calpains may possibly be different among these different conditions. Indeed, it is likely that Ca 2+ influx though N- methyl- D -aspartate receptors and other Ca 2+ sources may have a central role in TDP-43 mislocalization in ischaemic and traumatic brain injury. Although pathogenic roles of endoplasmic reticulum stress and mitochondrial damage are implied in ALS [47] , [48] , a role for internal Ca 2+ storage vesicles in TDP-43 pathology, however, has not been demonstrated. TDP-43 pathology is rarely, if ever, observed in the motor neurons of patients with SOD1 -associated ALS or in SOD1 Tg animals [24] , [49] . We found different expression profiles of calpains and CAST in our AR2 mice and SOD1 Tg mice. There was a marked upregulation of calpain without a change in CAST in AR2 mice ( Supplementary Fig. S4 ), in contrast to the decreased expression levels of calpains and an increase in CAST and cleaved forms of CAST in SOD1 Tg mice [50] , [51] , [52] . The difference between these two ALS model lines suggests a mechanistic difference between SOD1 -associated ALS and sporadic ALS. At present, it is unclear whether neurodegeneration results from a loss of TDP-43 function in the nucleus or a toxic gain-of-function effect from cytosolic sequestration. The results from Tg mice expressing wild-type human and mouse TDP-43 are consistent with respect to the loss of nuclear TDP-43 but not cytoplasmic mislocalization [1] , [35] , [53] , [54] . In addition to generating aggregation-prone fragments, the cleavage of TDP-43’s C-terminal disrupts binding to hnRNP A1, histone deacetylase 6 and fused in sarcoma/translocated in liposarcoma [2] , [55] , [56] . How neurons bearing TDP-43 pathology undergo neuronal death remains to be elucidated, but the present results on AR2 and AR2H mice indicate that the motor neurons expressing Q/R site-unedited GluA2 (refs 18 , 25 ) exhibit loss of TDP-43 in the nucleus but not necessarily abnormal cytoplasmic inclusions during the process to death. Given the potentially deleterious effects of TDP-43 pathology, the calpain-mediated TDP-43 cleavage pathway may serve as a therapeutic target for ALS and other neurological diseases exhibiting TDP-43 pathology. In vitro translation To generate full-length TDP-43 expression constructs, we first amplified the TDP-43 coding region from human HeLa cell line cDNA using the following primers: TDP-43UP1, 5′-AAAAAAACGCGTGCCGCCATGTCTGAATATATTCGGGTAACCG-3′ and TDP-43DW1; 5′-TATTACGCGTCTACATTCCCCAGCCAGAAGACTTAG-3′. After gel purification, PCR products were digested with Mlu I and inserted into the pTNT vector (Promega, Madison, WI, USA), then digested with the same restriction enzyme. Mutant TDP-43 cDNAs with the A315T and M337V mutations were prepared by site-directed mutagenesis and cloned into the pTNT vector. The production of recombinant TDP-43 proteins by in vitro translation was carried out using a TNT T7 Quick Coupled Transcription/Translation System (Promega). Construction of plasmids To construct N-terminally GFP-fused TDP-43 (pEGFP-C3-TDP-43), pEGFP-C3-TDP-43 fragments (1–243, 1–286, 1–324, 324–414), C-terminally GFP-fused TDP-43 (pEGFP-N2-TDP-43) and N-terminally His 6 -tag-fused TDP-43 (TDP-43-pCold I), a cDNA encoding full-length TDP-43 was amplified from pTNT-TDP-43 using the following primers: GFP-C3-forward, GFP-C3-reverse, TDP1-243-reverse, TDP1-286-reverse, TDP1-324-reverse, TDP324-414-forward, GFP-N2-forward, GFP-N2-reverse, HIS-N-forward and HIS-N-reverse ( Supplementary Table S3 ). The amplified fragment was digested with Xho I /Bam HI or Kpn I /Xho I and cloned into the same cleavage sites of the pEGFP-C3 vector (Clontech) and pCold I vector (Takara). Site-directed mutagenesis of His 6 -tagged or non-tagged full-length TDP-43 was carried out to substitute Ala315 to Thr (A315T), Met337 to Val (M337V), Ile 318 to Arg (I318R) using a KOD Plus mutagenesis kit (Toyobo). Cell culture and transfection Neuro2a and HeLa cells were cultured in DMEM high-glucose medium (Wako, Tokyo, Japan) supplemented with 10% foetal bovine serum (Invitrogen, Carlsbad, CA, USA), 100 U ml−1 penicillin and 100 μg ml −1 streptomycin (Invitrogen), in 5% CO 2 at 37 °C. HeLa cells were transfected using Lipofectamine LTX and PLUS reagents (Invitrogen). The cells were cultured for 72 h and were then collected. Human autopsy material Frozen brains and spinal cords that had been obtained at autopsy from patients with sporadic ALS including those with ALS with dementia (FTLD-MND; n =4) and from control subjects free from neurological diseases ( n =3) maintained at −80 °C were used. Consent for autopsy and approval for the use of tissue specimens for research purposes was obtained from the patients before death. Animals The mutant animals used in this study were homozygous ( ADAR2 flox/flox /VAChT-Cre.Fast; AR2) [18] and heterozygous ( ADAR2 flox/+ /VAChT-Cre.Fast; AR2H) conditional ADAR2 knockout mice [25] , AR2res ( ADAR2 flox/flox /VAChT-Cre.Fast/GluR-B R/R ) mice [18] , CAST Tg [28] and knockout (CAST KO) mice [27] . AR2res ( ADAR2 flox/flox /VAChT-Cre.Fast/GluR-B R/R ) mice were generated by crossbreeding AR2 mice with GluR- B R/R mice in which the endogenous GluA2 gene ( Glia2 ) were engineered to encode directly edited GluA2, and ADAR2-lacking motor neurons did not undergo neuronal death by 6 months of age [18] , [25] . CAST Tg and CAST KO mice were bred as described previously [27] , [28] . Wild-type mice of the same strain at the same age were used for the controls. The Committee on Animal Handling at the University of Tokyo approved all experimental procedures used. In vitro calpain and caspase assays Neuro2a and HeLa cells were homogenized by sonication in ten volumes of extraction buffer (50 mM HEPES, pH 7.5, 1 mM EDTA, 100 mM NaCl, 10 mM dithiothreitol (DTT) and 0.1% CHAPS). The homogenate was centrifuged at 1,000 g for 10 min at 4 °C. The supernatant was incubated at 30 °C with 0.5–5.0 units of purified human erythrocyte μ-calpain (calpain-I) or 3.0–30 units recombinant human caspase-3 in extraction buffer, with or without 5 mM CaCl 2 . The reaction was stopped by addition of SDS sample buffer containing 62.5 mM Tris–HCl, pH 6.8, 4% SDS, 10% glycerol, 50 mM DTT and 0.1% bromophenol blue. The samples were boiled at 100 °C for 5 min. Fifty microliters of the recombinant TDP-43 or mutant TDP-43 protein, which were synthesized by the TNT T7 Quick Coupled Transcription/Translation Systems, were homogenized by sonication in 450 μl of extraction buffer (5 mM cysteine and 150 mM imidazole, pH 7.5) [57] . The homogenate was centrifuged at 1,000 g for 10 min at 4 °C. The supernatant was incubated at 30 °C with 0.2–0.5 units of purified human erythrocyte μ-calpain (calpain-I) or 0.5 units of purified porcine kidney m-calpain (calpain-II) in extraction buffer, with or without 5 mM CaCl 2 . The SDS sample buffer (62.5 mM Tris–HCl, pH 6.8, 4% SDS, 10% glycerol, 50 mM DTT and 0.1% bromophenol blue) was added to stop the reaction, and the sample was boiled at 100 °C for 5 min immediately before SDS–PAGE analysis. Analysis of calpain activity in mice brain and spinal cord For in vitro TDP-43 cleavage experiments, the whole brains or the spinal cord of the mice at 7 months of age were homogenized in tenfold volumes of extraction buffer (5 mM cysteine and 150 mM imidazole, pH 7.5) and the supernatant of centrifugation at 18,000 g for 20 min was used as brain or spinal cord extracts. The cleavage of TDP-43 was induced by incubation of the extracts in the presence of 5 mM CaCl 2 at 30 °C (ref. 58 ). The SDS sample buffer was added to stop the reaction. Protein extraction The samples, including frozen human and mouse brains and spinal cords, were homogenized in ten volumes of extraction buffer (0.25 M sucrose/TKM buffer (50 mM Tris–HCl buffer; pH 7.5)) containing 25 mM KCl, 5 mM MgCl 2 and 0.5 mM DTT) [59] . After the homogenate was centrifuged at 1,000 g at 4 °C for 10 min, SDS sample buffer was added and the sample was boiled at 100 °C for 5 min immediately before SDS–PAGE analysis. Sarkosyl-insoluble urea-soluble fraction of TDP-43 Sarcosyl-insoluble urea-soluble TDP-43 fraction was extracted using the method previously described [10] . Human brain samples were homogenized in ten volumes of extraction buffer (10 mM Tris–HCl, pH 7.5, 0.8 M NaCl, 5 mM EDTA, 1 mM EGTA, 10% sucrose, phosphatase inhibitor cocktail (Roche) and protease inhibitor cocktail (Pierce)), then spun at 386,000 g for 20 min at 4 °C. The supernatant was recovered as the Tris-soluble fraction. The Tris-insoluble pellets were lysed in extraction buffer containing 1% (v/v) Triton X-100. The homogenates were left at 37 °C for 30 min and then centrifuged at 386,000 g at 4 °C for 20 min. After a 20-min spin at 386,000 g , the resultant supernatant was retained as a Triton-soluble fraction and the pellet was homogenized in extraction buffer containing 1% sarkosyl. The homogenate was incubated at 37 °C for 30 min and then subjected to a 20-min spin at 386,000 g . The resultant supernatant was retained as the sarkosyl-soluble fraction, and the pellet was solubilized in one volume of 50 mM Tris–HCl, pH 7.5, containing 8 M urea. This process was followed by a 20-min spin at 386,000 g . The supernatant was retained as the sarkosyl-insoluble, urea-soluble fraction. Immunohistochemistry Immunohistochemistry was performed as previously described by Hideyama et al . [18] Immunofluorescent staining of the sections was performed using rabbit anti-TDP-43 (ProteinTech Group Inc., 1:100) and sheep anti-rat RED1 (ADAR2; Exalpha Biologicals, Inc., 1:100) for the primary antibodies. Sections were then incubated with Alexa Fluor 488 donkey anti-sheep IgG (Invitrogen, 1:100) and Alexa Fluor 647 chicken anti-rabbit IgG (Invitrogen, 1:100), respectively, as the secondary antibodies. The sections were examined under an LSM-510 confocal microscope (Zeiss) after staining with 0.5 μM TO-PRO-3 for 30 min (ref. 10 ). Identification of calpain cleavage sites of TDP-43 The pCold I DNA construct inserted TDP-43 cDNA was transformed into chaperone competent cells BL21 Escherichia coli (Takara). Cells were grown in 10 ml LB containing Ampicillin (50 μg ml −1 ) L -arabinose (0.5 mg ml −1 ), Tetracycline (5 ng ml −1 ) and Chloramphenicol (20 μg ml −1 ) at 37 °C and induced with 1 mM isopropyl-β-d-thiogalactoside (Acros) at 15 °C for 24 h. Cells were collected by centrifugation at 1,000 g at 4 °C for 5 min. E. coli cells and HeLa cells resuspended in 1 ml of extraction buffer (50 mM HEPES, pH 7.5, 1 mM EDTA, 100 mM NaCl, 10 mM DTT and 0.1% CHAPS) containing protease inhibitors (Roche), and were homogenized by sonication. The supernatant was incubated at 30 °C with ten units of purified human erythrocyte μ-calpain (calpain-I) in extraction buffer with 5 mM CaCl 2 . The purification of recombinant polyhistidine-tagged proteins using TALON single columns (Takara) was performed following the user manual (Takara). The reaction was stopped by addition of SDS sample buffer containing 156 mM Tris–HCl, pH 6.8, 10% SDS, 25% glycerol, 30% 2-mercaptoethanol and 0.1% bromophenol blue. The samples were boiled at 100 °C for 10 min immediately before SDS–PAGE analysis. The purified proteins were stained with Bio-Safe Coomassie (Bio-Rad). Individual gel bands were then manually excised and subjected to overnight-automated digestion with sequencing grade modified trypsin at 35 °C. After desalting by using ZipTip C18 (Millipore), samples were mixed with a matrix, 2, 5-dihydroxybenzoic acid and allowed to air dry. MS was carried out on Voyager-DE STR (Applied Biosystems, USA). Peptide mass and corresponding MS/MS fragmentation information for each sample were searched against the His6-TDP-43 protein sequence using Mascot server version 2.2 (Matrix Science). Statistical analysis Average data are presented as means and s.e.m. Statistical analysis was carried out using the JMP 8 software (SAS Institute Inc.). For statistical comparison of two groups, we used unpaired, two-tailed Student’s t -test. Differences were considered significant when P <0.05. How to cite this article: Yamashita, T. et al . A role for calpain-dependent cleavage of TDP-43 in amyotrophic lateral sclerosis pathology. Nat. Commun. 3:1307 doi: 10.1038/ncomms2303 (2012).